Three-dimensional deep sub-diffraction optical beam lithography with 9 nm feature size The current nanofabrication techniques including electron beam lithography provide fabrication resolution in the nanometre range. The major limitation of these techniques is their incapability of arbitrary three-dimensional nanofabrication. This has stimulated the rapid development of far-field three-dimensional optical beam lithography where a laser beam is focused for maskless direct writing. However, the diffraction nature of light is a barrier for achieving nanometre feature and resolution in optical beam lithography. Here we report on three-dimensional optical beam lithography with 9 nm feature size and 52 nm two-line resolution in a newly developed two-photon absorption resin with high mechanical strength. The revealed dependence of the feature size and the two-line resolution confirms that they can reach deep sub-diffraction scale but are limited by the mechanical strength of the new resin. Our result has paved the way towards portable three-dimensional maskless laser direct writing with resolution fully comparable to electron beam lithography. While it is not a cost-effective solution, electron beam lithography (EBL) facilitates nanometre resolution [1] because of the diffraction nature of an electron beam that exhibits an extremely short De Broglie wavelength ( Fig. 1a ). Though the use of near-field nano-focusing has recently enabled low-cost plasmonic lithography with sub-100 nm resolution and 22 nm feature size [2] , this approach inherently cannot facilitate the nanofabrication of three-dimensional (3D) structures that are highly required in next-generation nanophotonic devices [3] , [4] . Optical beam lithography (OBL) based on focusing through a high numerical aperture objective [5] is an ultimate approach to 3D nanofabrication ( Fig. 1b ). However, the diffraction nature of light prevents us from achieving sub-diffraction or nanometre resolution in an OBL system [5] . Even for two-beam OBL based on the polymerization and photoinhibition strategy [6] , [7] , [8] , [9] , [10] , it has been impossible to realize the fabrication with feature size and resolution comparable to that achievable by EBL due to the lack of photoresins with large two-photon absorption cross-section, high mechanical strength and sufficient photoinhibition function. 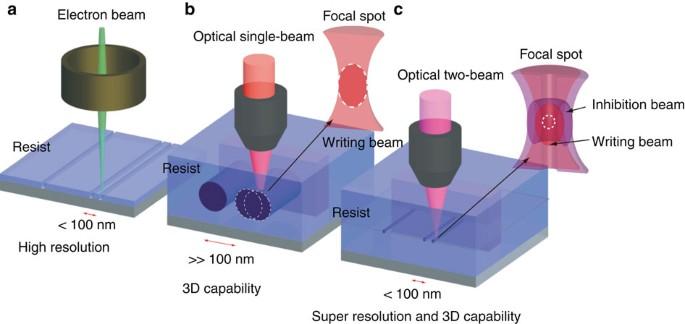Figure 1: Comparison of different lithography schemes. (a) EBL can achieve high resolution of ~10–20 nm; however, EBL is incapable of 3D fabrication. (b) Single-beam OBL can fabricate 3D arbitrary geometry; however, the diffraction nature of light limits fabrication resolution. (c) Two-beam OBL has the advantage of fabricating 3D arbitrary geometry with nanometer feature size and resolution comparable to EBL by the photoinhibition strategy. The image in the inset shows the focal spot of the writing beam and the inhibition beam. Figure 1: Comparison of different lithography schemes. ( a ) EBL can achieve high resolution of ~10–20 nm; however, EBL is incapable of 3D fabrication. ( b ) Single-beam OBL can fabricate 3D arbitrary geometry; however, the diffraction nature of light limits fabrication resolution. ( c ) Two-beam OBL has the advantage of fabricating 3D arbitrary geometry with nanometer feature size and resolution comparable to EBL by the photoinhibition strategy. The image in the inset shows the focal spot of the writing beam and the inhibition beam. Full size image Compared with single-beam OBL, two-beam OBL utilizes a doughnut-shaped inhibition beam to inhibit the photopolymerization triggered by the writing beam at the doughnut ring, leading to reduced feature size and improved resolution ( Fig. 1c ). Although both focused writing and inhibition beams result in the spot size limited by diffraction, the fabricated feature size and resolution by two-beam OBL can break the limit defined by the diffraction spot size of the two focused beams. In fact, the smallest feature size and the highest resolution are limited by the mechanical strength of the solidified material, which can be far beyond the diffraction limit provided that an appropriate photoresin with high mechanical strength can be developed. But this breakthrough has not yet been achieved. Here, we demonstrate 3D deep sub-diffraction OBL with 9 nm ( λ /42 for the wavelength of the inhibition beam) feature size and 52 nm ( λ /7) two-line resolution in a resin that can efficiently harness two-photon polymerization (2PP) and single-photon inhibition. Development of a new photoresin The key to 3D deep sub-diffraction OBL is the development of a unique material with two chemical activation channels. One is for photopolymerization and the other is for photoinhibition. For this aim, the material should be designed to satisfy the following requirements. First, it should include an initiator that is highly photosensitive to two-photon absorption generated by a writing beam, which allows for the near-threshold fabrication. Accordingly, it is possible to achieve a minimum degree of photopolymerization required for building solidified structures with a feature size smaller than the focal spot of the writing beam. Second, it should exhibit an effective inhibition of the 2PP process, which is achieved by a doughnut-shaped inhibition beam in a wavelength region different from the writing beam. The cross excitation between the writing and the inhibition beams, which means the excitation of the inhibitor by the writing beam or the excitation of the initiator by the inhibition beam, should be avoided. Third, the threshold intensity I th for the writing beam to generate 2PP should be as low as possible to avoid photodamage and uncontrolled thermal process. Fourth, it should exhibit the sufficient mechanical strength so that the structures fabricated at the near-threshold condition can survive during the wash-out developing process and withstand the unavoidable stress. A critical development of the new photoresin was the appropriate selection of a photoinitiator that satisfies conditions 1, 2 and 3. We chose 2,5-bis( p -dimethylaminocinn amylidene)- cyclopentanone (BDCC) ( Fig. 2a ), which is an example of the D-π-A-π-D class of non-linear dyes. We examined π-conjugated ketone derivatives of this class [11] , [12] , [13] capable of two-photon excitation. They have electron-donating diakylamino groups and carbonyl groups as the electron-withdrawing (acceptor) group that also allows hydrogen abstraction for subsequent initiation of free radical polymerization. Moreover, the length of the π-conjugated chain in between donor and acceptor parts allowed the tuning of the position of the absorption band into the visible region ( Fig. 2b , red curve) and led to the enhancement of the two-photon cross-section ( Fig. 2b , blue curve). The red-shifted absorption band of BDCC facilitated the inhibition process when tetraethylthiuram disulphide (TED, see Supplementary Fig. S1 ) was adopted as an ultraviolet inhibitor. It was evident that the absorption peak of BDCC was shifted to 511 nm from 360 nm of bis(4-(dimethylamino) phenyl)methanone (BDEP; Supplementary Fig. S2 ) or from 480 nm of 2,5-bis-[4-(dimethylamino)-benzylidene] -cyclopentanone (BDMA; Supplementary Fig. S3 ), which both had shorter lengths of π-conjugation. The corresponding 800 nm wavelength two-photon cross-section of BDCC was enhanced to 300 GM from 128 GM of BDEP or from 225 GM of BDMA. In the meantime, the laser intensity threshold I th for 2PP with BDCC was reduced to 75.75 mW cm −2 from 303.03 mW cm −2 (BDEP) or from 189.39 mW cm −2 (BDMA) at the scanning speed of 160 μm s −1 . 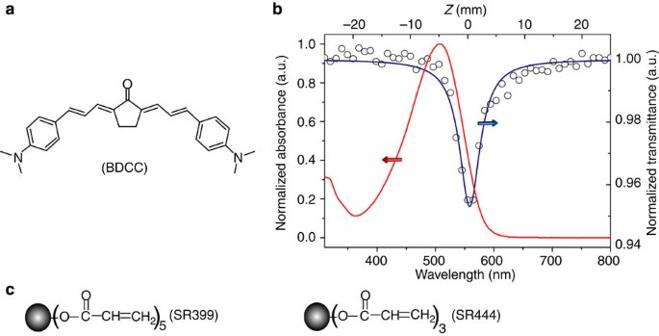Figure 2: Two-photon initiator and monomers. (a) The molecular structure of BDCC. The BDCC has the properties of low ultraviolet absorption and large two-photon absorption cross-section. (b) Single-photon absorption spectra of BDCC in chloroform and its two-photon cross-section obtained by the Z-scan method. (c) The monomers used in the photoresin are SR399, which has high functionality and can lead to fast curing, and SR444, which has low viscosity. Figure 2: Two-photon initiator and monomers. ( a ) The molecular structure of BDCC. The BDCC has the properties of low ultraviolet absorption and large two-photon absorption cross-section. ( b ) Single-photon absorption spectra of BDCC in chloroform and its two-photon cross-section obtained by the Z-scan method. ( c ) The monomers used in the photoresin are SR399, which has high functionality and can lead to fast curing, and SR444, which has low viscosity. Full size image For the selection of monomers, a five-functional monomer, SR399 (Dipentaerythritol pentaacrylate, Fig. 2c ), was used to improve the chemical reactivity for high photosensitivity and mechanical strength against the damage and the shrinkage ( Supplementary Fig. S4 and Supplementary Discussion ) during the developing process. Compared with other less-functional monomers, this five-functional monomer can provide a higher crosslinking density to reduce the gelation threshold and increase the mechanical strength for a given photopolymerization monomer conversion. Another trifunctional monomer, SR444 (pentaerythritol triacrylate, Fig. 2c ), was introduced to keep the viscosity from decreasing the photoinhibition efficiency. These two multi-functional monomers support sufficient gelation with the intensity of the writing beam below the level of the photodamage and the unwanted thermal process. With a standard initiation system of camphorquinone (CQ) and ethyl 4-(dimethylamino)benzoate (EDAB) as co-initiator, the photosensitivity of the final photoresin (see ‘Material synthesis’ in Methods) was confirmed to be at 0.18 g J −1 , implying at least two orders of magnitude higher than that of the formulation used in the single-photon fabrication [9] . Feature size reduction with 3D deep sub-diffraction OBL With our new two-photon absorption resin, which facilitates an immediate threshold operation ( Fig. 3a ), the 800-nm wavelength laser beam (see ‘Experimental setup’ in Methods and Supplementary Fig. S5 ) can produce not only a dot size of 95 nm (not shown here) but also the free-standing nanowires. Without the inhibition beam, the feature size, that is, the linewidth of the free-standing nanowire ( Supplementary Fig. S6 ) could be reduced from 150 nm (the black point in Fig. 3b ) to 42 nm (point A in Fig. 3b ), when the writing beam-dosed energy was decreased from 8 E min to E min (There exists a minimum energy dose E min for maintaining the fabricated polymer feature against destructive forces. Here, the E min is the experimentally observed minimum energy dose required to survive the fabricated free-standing nanowires). The smallest nanowire linewidth of 42 nm (point A in Fig. 3b ) was achieved in our new resin at the writing energy of E min . A further decrease of the writing beam energy dose decreased the degree of photopolymerization at the focal centre, leading to the disintegration of the fabricated structures after the developing process. This result indicates a critical limitation in the OBL due to the existence of the material threshold in the focal centre, resulting from the minimum monomer conversion required to compete with deconstructive forces, such as the change of the surface tensions. 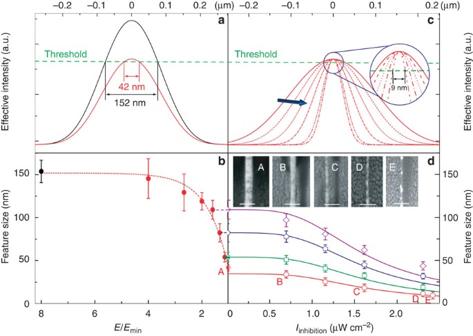Figure 3: Feature size measurement. (a) Schematic demonstration of the feature size reduction in single-beam OBL by decreasing the writing laser beam energy dose to the polymerization degree threshold of the photoresin. The black curve corresponds to the black point inb. The red curve corresponds to the point A inb. (b) Feature size versus the writing laser beam energy dose for the new resin without the inhibition beam in the experiment. (c) Schematic illustration of feature size reduction in two-beam OBL by increasing the intensity of the inhibition beam. The effective focal spot profile becomes narrower by increasing the intensity of the inhibition laser beam with the fixed irradiation intensity of the writing beam. The blue arrow suggests the direction of increasing the intensity of the inhibition laser beam. (d) Feature size of free-standing lines versus the intensity of the inhibition beam, under the exposure of the writing beam with different energy doses. The dots with error bars represent the experimental results. Curves guiding the dots are the fitting with the formula:. The insert pictures show the scanning electron microscopy images of points A, B, C, D and E with a scale bar of 100 nm. All the error bars reflect s.d. Figure 3: Feature size measurement. ( a ) Schematic demonstration of the feature size reduction in single-beam OBL by decreasing the writing laser beam energy dose to the polymerization degree threshold of the photoresin. The black curve corresponds to the black point in b . The red curve corresponds to the point A in b . ( b ) Feature size versus the writing laser beam energy dose for the new resin without the inhibition beam in the experiment. ( c ) Schematic illustration of feature size reduction in two-beam OBL by increasing the intensity of the inhibition beam. The effective focal spot profile becomes narrower by increasing the intensity of the inhibition laser beam with the fixed irradiation intensity of the writing beam. The blue arrow suggests the direction of increasing the intensity of the inhibition laser beam. ( d ) Feature size of free-standing lines versus the intensity of the inhibition beam, under the exposure of the writing beam with different energy doses. The dots with error bars represent the experimental results. Curves guiding the dots are the fitting with the formula: . The insert pictures show the scanning electron microscopy images of points A, B, C, D and E with a scale bar of 100 nm. All the error bars reflect s.d. Full size image While a doughnut-shaped inhibition beam is introduced into two-beam OBL ( Supplementary Fig. S5 ), the photoinhibition process is activated to confine the photopolymerization to the centre of the focal spot through the photo-excitation of the inhibitors (TED). As the inhibition process is achieved immediately near the threshold of the new material while the intensity of the writing beam at the focal centre remains the same as if there was no inhibition beam, the effective intensity profile (that is, the effecive focal spot size), equavalent to the area with the photopolymerization degree above the threshold becomes smaller ( Fig. 3c ). Thus, the photopolymerized feature size can be further reduced ( Fig. 3c ). As the photopolymerization is inhibited only in the ring of the doughnut-shaped inhibition beam in this method, the degree of the photopolymerization monomer conversion at the focus centre does not change and remains above the threshold, allowing the photopolymerized structure to survive after the developing process. With the inhibition beam of intensity levels of 0.69, 1.15, 1.62, 2.31 and 2.42 μW cm −2 , the feature size, that is, the linewidth of the free-standing nanowires is experimentally reduced from 42 nm (point A in Fig. 3d ) to 34 nm (point B in Fig. 3d ), 18 nm (point C in Fig. 3d ), 11 nm (point D in Fig. 3d ) and 9 nm (point E in Fig. 3d ), respectively, which agrees with the prediction by the theoretical numerical simulation ( Supplementary Fig. S7 ). The experimental and numerical simulation data can be fitted with a formula ( Supplementary Discussion [9] , [14] , [15] , [16] , [17] ): line width (nm) = with α 1 =34.48 (nm), β 1 = 0.44 ((μW cm −2 ) −3 ) and I S defined as the inhibition beam saturation intensity. The α 1 value varies as the inhibition beam applied at different energy dose of the writing beam (as shown in Fig. 3d ). The fabrication of lines with width below 50 nm using higher energy dose of the writing beam and higher inhibition beam intensity implies a large flexibility of the exposure latitude of the two beams, which greatly differs from single-beam OBL requiring critical exposure dose for obtaining small feature structures. A further analysis shows that the size dependence determined by with two-beam OBL holds in the axial direction ( Supplementary Fig. S8 and Supplementary Disscussion ). Resolution improvement with 3D deep sub-diffraction OBL Fabrication resolution is a different concept from feature size studied in Fig. 3 and can be determined by two-line resolution, which is the minimum centre-to-centre distance between the two fabricated lines. Though the condition for reducing the feature size is the necessary but not the sufficient condition for improving resolution, the realization of 9 nm feature size in two-beam OBL provides the prerequisite for the fabrication with the two-line resolution beyond the diffraction limit of the writing beam, as shown schematically in Fig. 4a . Without the inhibition beam, the two-line resolution achieved in the experiment is 246 nm (point A in Fig. 4b ), which is approximately the diffraction limit of the writing beam at the wavelength of 800 nm. 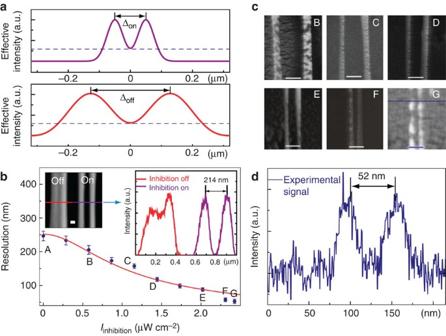Figure 4: Two-line resolution measurement. (a) Schematic demonstration of the two-line resolution improvement. Δonand Δoffrepresent the two-line resolution with and without the inhibition laser beam, respectively. The dashed line indicates the threshold of the effective intensity. (b) Two-line resolution versus the intensity of the inhibition laser beam. The inserted scanning electron microscopy (SEM) image shows two adjacent lines fabricated with the inhibition laser beam switched off and on, respectively. The insert is the plot of the cross-sectional profile of the inserted SEM image. The error bars reflect s.d. (c) SEM images of points B, C, D, E, F and G shown inb. (d) The cross-sectional profile of image G inc. Scale bars, 100 nm. Figure 4: Two-line resolution measurement. ( a ) Schematic demonstration of the two-line resolution improvement. Δ on and Δ off represent the two-line resolution with and without the inhibition laser beam, respectively. The dashed line indicates the threshold of the effective intensity. ( b ) Two-line resolution versus the intensity of the inhibition laser beam. The inserted scanning electron microscopy (SEM) image shows two adjacent lines fabricated with the inhibition laser beam switched off and on, respectively. The insert is the plot of the cross-sectional profile of the inserted SEM image. The error bars reflect s.d. ( c ) SEM images of points B, C, D, E, F and G shown in b . ( d ) The cross-sectional profile of image G in c . Scale bars, 100 nm. Full size image Breaking this resolution limit requires the photo-excitation of a sufficient quantity of photoinhibitors with the inhibition beam ( Supplementary Fig. S9 and Supplementary Disscussion ). The over-loading of photoinhibitors can compensate the loss of its concentration caused by the repeated scanning of the doughnut-shaped inhibition beam during the fabrication. As the intensity of the inhibition beam increases to 0.57, 1.15, 1.44, 2.02 and 2.31 μW cm −2 , accompanied with the decreasing linewidth, the resolution is improved from 246 nm to 205 nm (point B in Fig. 4b ), 157 nm (point C in Fig. 4b ), 117 nm (point D in Fig. 4b ), 87 nm (point E in Fig. 4b ) and 57 nm (point F in Fig. 4b ), respectively. The best resolution achieved is 52 nm (point G in Fig. 4b ) with an inhibition beam intensity of 2.42 μW cm −2 , which is 1/7 of the inhibition beam wavelength and 1/5 of the resolution as achieved without the inhibition beam, as shown in Fig. 4d . Fitting the experimental data (the red curve, which guides the blue experimental data in Fig. 4b ) reveals the resolution dependence on the inhibition intensity: resolution in-plane (nm)= with α 2 =252.07 (nm), β 2 =2.04 ((μW cm −2 ) −1 ). This dependence clearly shows that the resolution is far beyond the diffraction limit of the writing beam. In fact, the formula indicates the possibility of the fabrication resolution in the nanoscale. Compared with the dependence of the linewidth on the inhibition intensity, , revealed in Fig. 3 , the decrease rate of the two-line resolution is slower upon increasing the intensity of the inhibition beam, as is reflected by the different power indices of the inhibition beam intensity in the two formulas. This difference originates from the re-exposure of the photoresin for the fabrication of two adjacent lines, which requires higher intensity of the inhibition beam to suppress the polymerization in the space between these two lines than the single-line fabrication case. Further, fabricating more adjacent lines (in Fig. 5 ) can degrade the resolution as the exposure dose of the inhibition beam and the writing beam in a given region grows due to the repeated scans, which needs to restrain the polymerization between each line and compensate the consumption of photoinhibitors. With an inhibition beam intensity of 2.42 μW cm −2 , the resolution of 90 nm was realized for the fabrication of ten parallel lines ( Fig. 5c ). 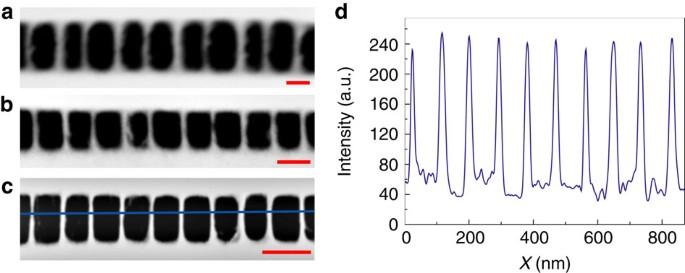Figure 5: Parallel free-standing nanowire fabrication. Scanning electron microscopy images of parallel free-standing nanowires fabricated under the exposure of the inhibition beam of 0.69 μW cm−2fora, 1.62 μW cm−2forb, 2.42 μW cm−2forc. Scale bars, 150 nm. (d) The graph shows the plot of the cross-sectional profile along the blue line inc. Figure 5: Parallel free-standing nanowire fabrication. Scanning electron microscopy images of parallel free-standing nanowires fabricated under the exposure of the inhibition beam of 0.69 μW cm −2 for a , 1.62 μW cm −2 for b , 2.42 μW cm −2 for c . Scale bars, 150 nm. ( d ) The graph shows the plot of the cross-sectional profile along the blue line in c . Full size image As for the two-line resolution in the z direction, a similar variation trend was revealed with increasing the intensity of the inhibition beam ( Fig. 6 ). The two-line resolution dependence on the inhibition intensity is fitted as: resolution in the z direction (nm)= , with α 3 =319.76 nm and β 3 =1.46 ((μW cm −2 ) −1 ). The β value is less than that for the in-plane direction, which indicates a reduced inhibition rate. This feature can be attributed to the inhibition process arising from the diffusion of the inhibitor radicals generated by the inhibition beam, since the inhibition beam with the in-plane doughnut shape cannot provide the direct inhibition function in the z direction. As the inhibition intensity increases to 2.42 μW cm −2 , the resolution is improved to 80 nm ( Fig. 6b ). 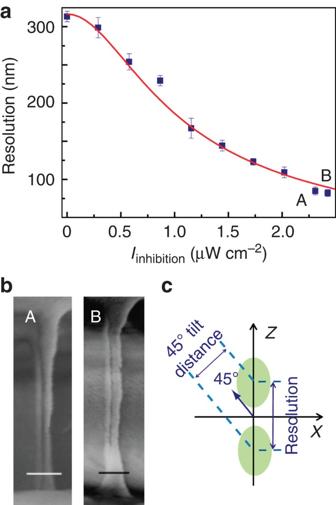Figure 6: Axial two-line resolution. (a) The graph shows the resolution variation as a function of the intensity of the inhibition beam. The error bars reflect s.d.. (b) The two scanning electron microscopy images correspond to two sets of the adjacent lines fabricated with the inhibition beam at the intensity of 2.31 μW cm−2and 2.42 μW cm−2, respectively. Scale bars, 200 nm. (c) Axial two-line resolution was obtained by viewing the sample tilted with 45° to the horizontal plane. Figure 6: Axial two-line resolution. ( a ) The graph shows the resolution variation as a function of the intensity of the inhibition beam. The error bars reflect s.d.. ( b ) The two scanning electron microscopy images correspond to two sets of the adjacent lines fabricated with the inhibition beam at the intensity of 2.31 μW cm −2 and 2.42 μW cm −2 , respectively. Scale bars, 200 nm. ( c ) Axial two-line resolution was obtained by viewing the sample tilted with 45° to the horizontal plane. Full size image The two-beam OBL method has led to the smallest feature size of 9 nm and the finest two-line resolution of 52 nm, which have never been achieved in OBL. The results shown in this paper indicates the feasibility of applying far-field optics to 3D nanofabrication ( Supplementary Fig. S10 ). With conventional optical and laser elements, this technology also enables low-cost and portable systems. Material synthesis For the realization of 3D deep sub-diffraction OBL with nanometre feature size and feature resolution, three two-photon photoinitiators, BDEP, BDMA and BDCC were introduced into the formulation [9] . The BDEP, known as Michler’s ketone, was purchased from Sigma-Aldrich and used as supplied. The synthesis of the BDMA was performed using a general method as outlined in the literature [18] . Lithium hydroxide monohydrate (0.1 ME, 28 mg, 0.671 mmoles) was added to cyclopentanone (1 ME, 0.564 g, 6.71 mmoles) in ethanol (12 ml) and stirred for 10 min. Then p-( N , N -dimethylamino)-benzaldehyde (2 ME, 2 g, 13.4 mmoles) was added and the reaction was stirred overnight. The reaction was worked up by dilution with ethanol and collection by filtration. The material was recrystallized from chloroform (ca. 150 ml for 3 g) to give 0.65 g. The mother liquor was evaporated to half the initial amount and another 0.85 g was harvested. Both batches were of the same high purity. 1 H NMR (CDCl 3 , 400 MHz) δ 3.03 (s, 6H, CH 3 ), 3.07 (s, 4H, CH 2 ), 6.73 (d, 2H, aromatic J 8.7 Hz), 7.52 (s, 2H, =CH-), 7.55 (d, 2H, aromatic, J 8.7 Hz) p.p.m. The synthesis of the BDCC was performed using a method similar to that used for the BDMA [9] . Lithium hydroxide monohydrate (0.1 ME, 28 mg, 0.671 mmoles) was added to cyclopentanone (1 ME, 0.564 g, 6.71 mmoles) in ethanol (12 ml) and stirred for 10 min. Then N , N -dimethylaminocinnamaldehyde (2.34 g, 13.4 mmoles, 2 ME) was added and the reaction was stirred for about 1 h with a dark red precipitate quickly forming. The reaction was worked up by dilution with ethanol and collection by filtration. The product was washed with ethanol and dried to give a dark brick red powder (2.3 g, 86%) 1 H NMR (CDCl 3 , 400 MHz) δ 2.86 (s, 4H, CH 2 ), 3.01 (s, 6H, CH 3 ), 6.66 (d, 2H, aromatic J 8.9 Hz), 7.75 (dd, 2H =CH, J 11.4 Hz 15.2 Hz), 6.88 (d, 2H, =CH, J 15.2 Hz), 7.23 (d, 2H, =CH-, 11.7 Hz), 7.38 (d, 2H, aromatic, J 8.7 Hz) p.p.m. The BDEP, BDMA and BDCC have two-photon cross-sections of 128 GM ( Supplementary Fig. S2 ), 225 GM ( Supplementary Fig. S3 ) and 300 GM under the exposure of wavelength 800 nm, respectively. Among these initiators, BDCC exhibited the highest two-photon cross-section and low absorption potential under the exposure of the inhibition beam operating at a wavelength of 375 nm, it was selected for use in the formulation for the 3D sub-diffraction OBL based on the photoinhibited polymerization method. As for the photoinhibitor, TED was introduced to the formulation, which can generate inhibitor radicals to scavenge propagating and initiating radicals to inhibit the polymerization. The photoinhibitor was excited by an ultraviolet beam with a wavelength of 375 nm. To avoid the excitation of the photoinhibitor by the writing beam, the photoinhibitor had no single-photon absorption and two-photon absorption under the exposure of the writing beam with the wavelength of 800 nm. Supplementary Fig. S1 shows the absorption spectrum of the TED. To prepare the photoresin, the photoinitiator (BDCC), co-initiators (CQ and EDAB) and the photoinhibitor TED were firstly dissolved in chloroform and then mixed with the monomers. The mixture was kept in the oven at the temperature of 50 °C for 24 h to remove the chloroform. The final formulation of the photoresin was composed of 0.02 wt% BDCC, 0.5 wt% CQ and 0.75 wt% EDAB as photoinitiator components and 2.5 wt% TED as the photoinhibitor, and 96.23 wt% monomer blends of SR399 and SR444 (40:60 wt%) (Sartomer Inc.). The photoresin was baked at 60 °C for 10 min before fabrication. Samples used for the fabrication were prepared by sandwiching a drop of the photoresin between two cover slips separated by 60 μm with thick sticky tapes. Experimental setup and characterization Supplementary Fig. S5 shows the setup of the 3D sub-diffraction OBL fabrication system. A femtosecond (fs) laser (Coherent, chameleon, USA) with a wavelength of 800 nm was used as the writing beam operating at a repetition rate of 80 MHz with a 140-fs pulse width. After the beam expansion, the writing beam was introduced into a high numerical aperture objective (NA=1.4, Olympus). A continuous wave mode laser (Coherent-cube, USA) with a wavelength of 375 nm was adopted as the inhibition beam. The inhibition beam was expanded after going through a half wave plate. It was then modulated by a phase plate (vortex phase, RPC Photonics Inc., USA) [19] to generate a focus profile with a zero intensity at the centre in the focal region for spatially confined photopolymerization. Then, the inhibition beam was overlapped with the writing beam at a dichroic mirror and focused by the objective. The λ /4 wave plate was used to modulate the inhibition beam to a circular polarized beam. Confocal detector photomultiplier tubes were used for the alignment of the system and the overlapping of the two beams. The intensity of the two beams was measured before entering the objective with a writing beam size of 26.4 mm 2 and an inhibition beam size of 86.6 mm 2 . A charge-coupled device camera was used to monitor the fabrication. The exposure of the writing beam and the inhibition beam to the photoresin for super-resolved feature fabrication was simultaneous, which are controlled by two synchronized shutters. For the fabrication of single lines without the inhibition beam, the writing beam intensity was fixed at 75.75 mW cm −2 with a scanning speed from 20 μm s −1 to 160 μm s −1 with the increasing step of 20 μm s −1 . The exposure energy dose of the writing beam used as the variable in the x axis ( Fig. 3b ) was calculated by multiplying the intensity with the exposure time. For the case with the inhibition beam, the writing beam intensity was fixed at 75.75 mW cm −2 and the scanning speed was changed from 100 μm s −1 to 160 μm s −1 , respectively. The fabrication of two adjacent lines was performed with a writing beam intensity of 75.75 mW cm −2 and a scanning speed of 160 μm s −1 . The two lines were sequentially fabricated by moving the photoresin while the positions of both focal spots were fixed. The left line was fabricated first for two-line resolution fabrication. For all the lines, they were suspended between two frames as free-standing lines. The frames were about 3 μm high above the cover slip and the lines are 900 nm lower than the top surface of the frames. The frame was adhered with the cover slip. After fabrication, the cover slip without sample structures was mechanically taken off with care, and then the structures were rinsed with isopropanol for 5 min, then acetone for 2 s and then ethanol for 2 s. The fabricated structures were measured with a ZEISS Supra 40 VP Field Emission Scanning Electron Microscope (accelerating voltage of 3 kV was used for measuring the patterns obtained in two-beam OBL). Before the measurement, the sample was coated with a gold layer with the thickness of 5–6 nm for the single-beam OBL and 1-2 nm for the two-beam OBL. The size of the fabricated lines is measured based on its cross-sectional profile obtained from the scanning electron microscopy image ( Supplementary Fig. S6 ). The full width at two third maximum was used for conservative estimation. To measure the two-photon cross-section of the two-photon initiators, the Z-scan method was used [20] . A fs-pulsed laser beam (Spitfire, Spectra-Physics, USA) with the repetition rate of 1 KHz, the pulse width of 110 fs and the wavelength of 800 nm was used as the light source. A convex lens with the focal length of 250 mm was used to focus the laser beam into the sample. The sample solution was sandwiched in a quartz cell with the thickness of 1 mm. It was prepared by dissolving the BDEP, BDMA and BDCC in chloroform, respectively, with the concentration of 2 × 10 −4 M. Fabrication of parallel nanowires Compared with the fabrication of two adjacent lines, the fabrication of parallel nanowires undoes more repeated scanning. Figure 5a–c shows the ten free-standing nanowires fabricated under the exposure of the inhibition beam with the varied intensities and the writing beam with the fixed intensity of 75.75 mW cm −2 , at the scanning speed of 160 μm s −1 . With increasing the intensity of the inhibition beam from 0.69 μW cm −2 to 2.42 μW cm −2 , the resolution is improved from 200 nm to 90 nm. 3D fabrication Free-standing nanwires, which were generated by sub-diffraction OBL are the building blocks for 3D nanostructures. As illustrations, two structures were fabricated. Supplementary Fig. S10a shows three layers of nanowires and X-shaped junctions fabricated by using the new resin, realising the minimum feature size of 22 nm. Supplementary Fig. S10b demonstrates four-layer stacked nanowires with the smallest feature size of 26 nm. These structures were fabricated with the intensity of 2.42 μW cm −2 of the inhibition beam and the intensity of 75.75 mW cm −2 of the writing beam at the scanning speed of 160 μm s −1 . The structures built at different depths of the medium enable the vertical integration of nano-patterns with a scalable high density in the third dimension. How to cite this article : Gan, Z. et al. Three-dimensional deep sub-diffraction optical beam lithography with 9 nm feature size. Nat. Commun. 4:2061 doi: 10.1038/ncomms3061 (2013).